The surface barrier phenomenon at the loading of metal-organic frameworks Loading with guest molecules is a crucial step for most applications of porous materials. For metal-organic frameworks, which are one of the most intensely investigated classes of porous materials, the experimentally determined rate of mass transfer into the material may vary by several orders of magnitude for different samples of the same material. This phenomenon is commonly attributed to the presence of so-called surface barriers, which appear to be omnipresent but poorly understood. Here we quantitatively study this phenomenon with a quartz crystal microbalance, using well-defined, highly crystalline, epitaxially grown thin films of metal-organic frameworks as a model system. Our results clearly demonstrate that surface barriers are not an intrinsic feature of metal-organic frameworks, as pristine films do not exhibit these limitations. However, by destroying the structure at the outer surface, for instance by exposure to air or water vapour, surface barriers are created and the molecular uptake rate is reduced. Metal-organic frameworks (MOFs) [1] are an important class of nanoporous crystalline materials with several exclusive properties: large surface areas [2] , high diversity [3] , [4] and the ability to alter these properties over wide ranges in a rational manner [5] , [6] . MOFs already have many interesting applications, such as storing hydrogen [7] or greenhouse [8] gases and for gas separation [9] . In other areas, including catalysis [10] and sensor techniques [11] , the first applications of MOFs are emerging. A crucial factor in all of these applications is guest molecule loading. Mass transfer of the guest molecules is a critical parameter governing performance; for example, in gas separation, poor transfer rates result in low separation efficiencies. Despite its importance, the loading of MOF materials with guest molecules is poorly understood on a quantitative level, and the values of diffusion coefficients measured for different samples of the same material may differ by several orders of magnitude. A prominent example is the diffusion of hydrogen in MOF-5. Experimental values reported for the corresponding diffusion coefficient vary by four orders of magnitude, between 10 −5 m 2 s −1 (ref. 12 ) and 10 −9 m 2 s −1 (ref. 13 ). Even when restricting the comparison to results reported by the same group using the same synthesis procedure for the MOF material used in the studies, variations of three orders of magnitude are found for CO 2 in MOF-5 (diffusion coefficients of 10 −9 m 2 s −1 and 10 −12 m 2 s −1 (refs 14 , 15 )). Another example is shown in Fig. 1a,b , where dramatic differences were found in the uptake of cyclohexane by thin MOF films and powder MOFs of the same structure. Analysing the experimental data, the (effective) diffusion coefficient of cyclohexane is roughly 1,000 times (or three orders of magnitude) larger for the thin film than for the powder material. In the case of ferrocene infiltration from a hexane solution, these differences are smaller, but the diffusion coefficient between the thin film and the powder material still differs by a factor of 5. 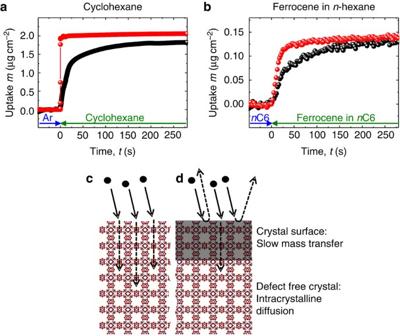Figure 1: Uptake by MOFs. The uptake of (a) cyclohexane (vapour) and (b) ferrocene from liquidn-hexane was significantly faster in thin HKUST-1 films (red, 150-nm thick) than in the corresponding powder material (black, ~200 nm crystal diameter, seeSupplementary Fig. 1). Uptake was determined using a quartz crystal microbalance24. (candd) Model of the mass transfer in MOFs. (c) Unhindered mass transfer in the nanoporous crystal. (d) Surface barriers hinder the guest molecules from entering the pore space and significantly slow down the mass transfer. Figure 1: Uptake by MOFs. The uptake of ( a ) cyclohexane (vapour) and ( b ) ferrocene from liquid n -hexane was significantly faster in thin HKUST-1 films (red, 150-nm thick) than in the corresponding powder material (black, ~200 nm crystal diameter, see Supplementary Fig. 1 ). Uptake was determined using a quartz crystal microbalance [24] . ( c and d ) Model of the mass transfer in MOFs. ( c ) Unhindered mass transfer in the nanoporous crystal. ( d ) Surface barriers hinder the guest molecules from entering the pore space and significantly slow down the mass transfer. Full size image First hints regarding the microscopic origin of these strong sample-to-sample variations have been provided by studies using interference microscopy [16] and infrared microimaging [17] . Analysis of intracrystalline concentration profiles found that so-called surface barriers may influence the uptake of molecules into these porous materials. These surface barriers, which act as additional mass transfer resistance at the outer crystal surfaces ( Fig. 1c ), hinder the molecules from entering and leaving the pores [18] , [19] . Although these barriers often dominate the entire mass transfer, particularly in the case of small powder particles, the underlying mechanism is, at best, qualitatively understood. In addition, whether all MOFs exhibit surface barriers and whether these barriers are an intrinsic feature of the material is unknown. Qualitatively, these surface barriers can be described as a thin layer with (reduced) permeability covering the external crystal surface [20] , [21] . To a good approximation, the uptake by a thin film, m ( t ), can be described by an exponential decay function: with a time constant of where l denotes the film thickness, D is the (transport) diffusivity, α is surface permeability, m eq the equilibrium loading and t the time. On the basis of equation (2), the uptake time increases quadratically with film thickness in the case of (bulk) diffusion-limited uptake processes. However, for surface barrier-limited uptake processes, the uptake time increases linearly with film thickness. Furthermore, the relative influence of the surface barrier on overall uptake increases with decreasing film thickness. Thus, the uptake of thin MOF films should be studied as a function of their thickness. A quantitative analysis of these results would allow more detailed insights into the microscopic origins of these surface barriers. Here we use surface-mounted MOFs (SURMOFs) of different thicknesses to quantitatively analyse the importance of surface barriers. SURMOFs are highly crystalline, oriented, thin MOF films grown by liquid-phase epitaxy on solid substrates in a well-defined layer-by-layer manner [22] . Suitable functionalization of the substrate is required for nucleating SURMOF growth on the substrate surface and controlling crystal orientation. Under adequate conditions, SURMOFs grow uniformly and film roughness as low as the size of a MOF unit cell can be achieved [23] . Apart from many potential applications, including chemical sensors and membranes, SURMOFs are well suited for a quantitative analysis of dynamic phenomena within MOFs [24] , [25] , [26] . In the present study we used HKUST-1, which is also known as Cu 3 (BTC) 2 , MOF-199 or Basolite C300 (ref. 27 ). HKUST-1 is one of the most popular MOFs [28] , [29] and is among the few that are commercially available [30] . HKUST-1 has a three-dimensional, isotropic pore space of big cages that are connected by 0.9-nm-diameter windows [27] , [31] . In addition to the large pores, the material has small side pockets with 0.46-nm-diameter windows. Cyclohexane is used as a prototype guest molecule. It has a kinetic diameter of ~0.6 nm [32] and the small side pockets are not accessible. Uptake by pristine HKUST-1 SURMOFs of varying thicknesses A quartz crystal microbalance (QCM) was employed to synthesize the HKUST-1 SURMOF in a clean and well-controlled manner and to perform the uptake experiments. The QCM sensor was placed in a flow cell (Q-Sense E4). Infiltration with guest molecules was achieved via a flow of gas or a stream of liquid through the cell [25] . The SURMOF to be investigated was grown directly on the gold-coated QCM sensor after functionalization with a 16-mercaptohexadecanoic acid self-assembled monolayer (MHDA SAM). SURMOF growth was carried out in situ in the QCM flow cell by alternating between the metal source solution (1 mM copper(II) acetate), a solution of 0.2 mM 1,3,5-benzenetricarboxylic acid (BTC) in ethanol and pure ethanol as described previously [33] . Not only does this synthesis procedure allow study of the growth process in situ , it also guarantees that the sample is never exposed to any environmental contaminants, such as humid air. Such contaminants are external factors that might affect the crystal structure. In addition to the clean synthesis in the flow cell, synthesis in the QCM cell enables an exact determination of the SURMOF mass by applying the Sauerbrey equation [34] ( Fig. 2 ). The structures of the SURMOF thin films grown on the QCM substrates were monitored by ex situ X-ray diffraction (XRD; see Supplementary Fig. 2 ). 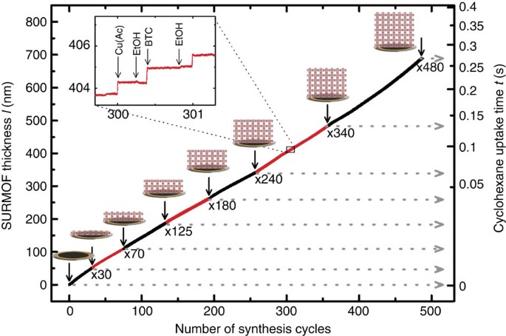Figure 2: Layer-by-layer growth of the HKUST-1 SURMOF on the QCM sensor. The synthesis was interrupted after 30, 70, 125, 180, 240, 340 and 480 cycles to perform uptake experiments with the probe molecule cyclohexane. The inset is a magnification of the layer-by-layer growth of the SURMOF. The left scale shows the quadratic increase in the uptake time of the probe molecule with increasing film thickness. Figure 2: Layer-by-layer growth of the HKUST-1 SURMOF on the QCM sensor. The synthesis was interrupted after 30, 70, 125, 180, 240, 340 and 480 cycles to perform uptake experiments with the probe molecule cyclohexane. The inset is a magnification of the layer-by-layer growth of the SURMOF. The left scale shows the quadratic increase in the uptake time of the probe molecule with increasing film thickness. Full size image Using this approach, the loading of cyclohexane by thin MOF films of specific thicknesses was studied ( Fig. 3 ). The cyclohexane loading relative to the SURMOF mass was found to be independent of the SURMOF thickness ( Fig. 3a ), showing that the SURMOF is homogenous. A relative cyclohexane loading of ~0.26 g cyclohexane per 1 g (activated) HKUST-1 was determined, which corresponds to a capacity of 33 cyclohexane molecules per HKUST-1 unit cell. The time-dependent uptake curves ( Fig. 3b and Supplementary Fig. 3 ) were used to determine the quantitative mass transfer into the thin SURMOF films. The time constants of the uptake processes were determined by fitting the experimental data with equation (1), resulting in reasonable fits (see Supplementary Fig. 3 ). The time constant of uptake versus film thickness ( Fig. 3c ) revealed a clear quadratic increase in uptake time with increasing film thickness. This observation directly shows that the mass transfer of cyclohexane into the HKUST-1 SURMOF is not influenced by surface barriers, but it is almost exclusively determined by intracrystalline diffusion. This was also demonstrated by plotting the normalized uptake versus the normalized time (that is, time divided by the square of the film thickness), resulting in coinciding plots ( Fig. 3d ). By using equation (2) and neglecting the surface barriers, the cyclohexane diffusivity was determined to be 6 × 10 −13 m 2 s −1 ( Fig. 3c ). 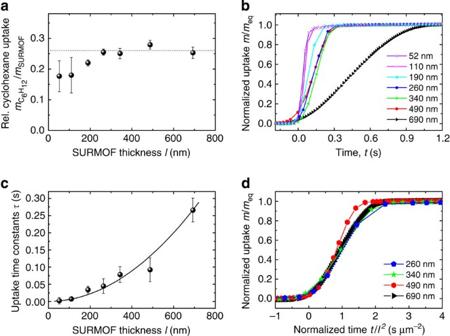Figure 3: Cyclohexane uptake. (a) Cyclohexane loading relative to the mass of the HKUST-1 SURMOF. The relative cyclohexane loading was unaffected by the SURMOF thickness. The dotted line represents the average value of 0.26 g g−1. (b) Normalized cyclohexane uptake for varying film thicknesses. The uptake rate slowed down with increasing film thickness. The inset shows the SURMOF thicknesses. (c) Time constants for cyclohexane uptake. The time constant for cyclohexane uptake increased quadratically with increasing SURMOF thickness. The black line isτ=l2/DwithD=6 × 10−13m2s−1. (d) Normalized uptake as a function of normalized time (that is, time divided by the square of the film thickness). The error bars ina,crepresent the s.d.’s of the experimental results. Figure 3: Cyclohexane uptake. ( a ) Cyclohexane loading relative to the mass of the HKUST-1 SURMOF. The relative cyclohexane loading was unaffected by the SURMOF thickness. The dotted line represents the average value of 0.26 g g −1 . ( b ) Normalized cyclohexane uptake for varying film thicknesses. The uptake rate slowed down with increasing film thickness. The inset shows the SURMOF thicknesses. ( c ) Time constants for cyclohexane uptake. The time constant for cyclohexane uptake increased quadratically with increasing SURMOF thickness. The black line is τ = l 2 / D with D =6 × 10 −13 m 2 s −1 . ( d ) Normalized uptake as a function of normalized time (that is, time divided by the square of the film thickness). The error bars in a , c represent the s.d.’s of the experimental results. Full size image From the data in Fig. 3c , we estimated a lower limit of surface permeability, that is, the maximum influence of the surface barrier. Using τ >> τ surface−barrier = l / α , we obtained a lower limit of ~10 −5 m s −1 for surface permeability α . As the relative influence of the surface barriers decreased with increasing crystal size, we concluded that surface barriers have vanishing influence on the mass transfer in pristine and defect-free MOF powders, which typically consist of large 1–100 μm crystals. Owing to the similarities in their pore spaces, this conclusion can probably be generalized to most MOF structures. Origin of surface barriers In order to obtain a better understanding of what causes surface barriers in MOFs, the thin MOF films, which exhibited no evidence of surface barriers, were modified using different procedures ( Fig. 4 ). A pristine SURMOF was immersed for 10 min in the solution (0.15 M copper(II)acetate and 0.1 M BTC in pure ethanol) used for the solvothermal synthesis of powder HKUST-1 MOFs. An increase in mass was observed (see Supplementary Fig. 4 ), indicating that MOF crystallites grew on top of the SURMOF film. Cyclohexane uptake by this sample was greater than the uptake by the SURMOF alone, and the uptake was also slightly slower (both by a factor of ~1.2, Fig. 4a ). However, a significant deceleration of the mass transfer was not observed. This observation provides strong evidence that surface barriers are not caused by the solvothermal synthesis conditions. 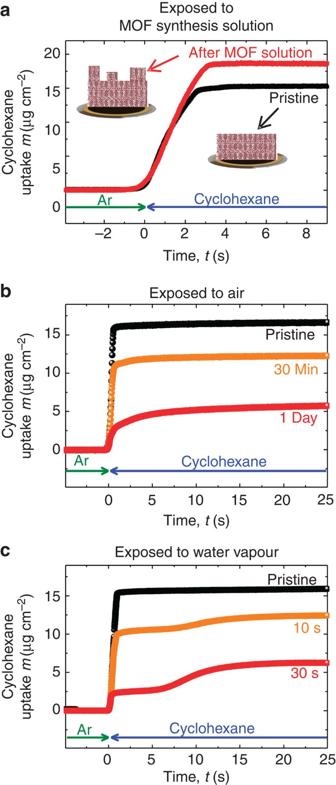Figure 4: Cyclohexane uptake after treatment of the thin MOF film. (a) The SURMOF was exposed to MOF synthesis solution and MOF crystallites grew on the SURMOF. Uptake by the SURMOF with MOF crystallites on top (red) was larger and marginally slower than the uptake by the pristine SURMOF (black). (b) Uptake by the SURMOF was significantly decreased and retarded by exposing the SURMOF to air for 30 min and 1 day. (c) Exposing the SURMOF to water vapour with a partial pressure of 23 mbar for 10 and 30 s at 30 °C caused a decrease in and significant deceleration of uptake. All three pristine SURMOF samples had a thickness of ~700 nm. Figure 4: Cyclohexane uptake after treatment of the thin MOF film. ( a ) The SURMOF was exposed to MOF synthesis solution and MOF crystallites grew on the SURMOF. Uptake by the SURMOF with MOF crystallites on top (red) was larger and marginally slower than the uptake by the pristine SURMOF (black). ( b ) Uptake by the SURMOF was significantly decreased and retarded by exposing the SURMOF to air for 30 min and 1 day. ( c ) Exposing the SURMOF to water vapour with a partial pressure of 23 mbar for 10 and 30 s at 30 °C caused a decrease in and significant deceleration of uptake. All three pristine SURMOF samples had a thickness of ~700 nm. Full size image The impact of environmental conditions was investigated by exposing a pristine SURMOF to air at 298 K and 30% relative humidity for 30 min. A decrease in the adsorption capacity and a significant deceleration of the uptake process were observed ( Fig. 4b ). After exposing the SURMOF to air for another 24 h, a further decrease in the adsorption capacity and mass transfer was observed. By exposing a pristine SURMOF to water vapour for only a short time (10 and 30 s), we showed that water is responsible for the decrease in and dramatic retardation of uptake ( Fig. 4c ). A quantitative analysis of the uptake curves in Fig. 4b,c) shows that, in both cases, the uptake rates decreased by a factor of ~30. Although exposure to water-containing air and water vapour had dramatic effects on mass transfer, the changes in crystallinity as monitored by XRD were minor (see Supplementary Fig. 5 ). Therefore, we concluded that exposure to water vapour mainly affects the crystal structure at the outer surface and not the bulk of the crystalline film, and that this destruction creates the surface barriers. One might generalize that water is responsible for causing surface barriers in all non-water-stable MOFs, the majority of MOFs. Previous studies [35] , [36] have shown that the transport resistance of surface barriers results from a total blockage of the pore entrances and that the uptake and release occurs by detours via unblocked pores, which remain fully opened. This means water molecules destroy the MOF structure close to the crystal surface, resulting in blocked pore entrances that have to be bypassed by the guest molecules during the mass transfer, causing the additional mass transfer resistance referred to as surface barriers. As a direct result of this model, the activation energy of the surface barrier equals the activation energy of the diffusion in the film. By using equation (2) and neglecting the diffusion term, the surface permeabilities α of both SURMOF films exposed to air or water vapour can be calculated to roughly 10 −7 m s −1 . By adapting equation (2) from ref. 35 to HKUST-1, which has an isotropic pore system, the fraction of open pore entrances p open can be calculated by p open =12 λ /5 × α / D , with λ denoting the distance between the pores (here: λ =1.3 nm [27] ), resulting in p open =0.05%. This means most of the pore entrances are blocked and only one out of 2,000 pore entrances remains open. In conclusion, the mass transfer in HKUST-1 MOFs was investigated in detail using thin, quasi-epitaxial grown films (SURMOFs) with different thicknesses and by studying the uptake of a prototype probe molecule, cyclohexane, using QCM. For pristine SURMOFs, the time for cyclohexane uptake increased quadratically with film thickness, indicating that the mass transfer is controlled by intracrystalline diffusion rather than by surface barriers. This observation demonstrates that, in contrast to common belief, surface barriers are not intrinsic properties of MOFs. Furthermore, exposing the MOF to air or water vapour creates surface barriers. Our results demonstrate that clean, particularly water-free, synthesis and storage are crucial for obtaining MOFs with high mass transfer rates. Synthesis of powder HKUST-1 MOF Powder HKUST-1 was solvothermally synthesized by mixing 0.30 g (1.5 mmol) copper(II) acetate and 0.21 g (1 mmol) BTC in 12 ml pure ethanol in a sealed glass bottle [37] . The reagents were mixed and dissolved in ultrasonic bath for 30 min, followed by heating at 65 °C for 2 days and cooling down to room temperature. The resulting powder was washed with pure ethanol and dried in nitrogen. By comparing with the simulated XRD of HKUST-1, the recorded XRD shows that powder HKUST-1 was synthesized ( Supplementary Fig. 1 ) [27] . Finally, powder HKUST-1 suspension in ethanol was prepared and spin-coated on the MHDA-functionalized QCM sensor. SURMOF synthesis and cyclohexane uptake experiments The HKUST-1 SURMOF synthesis was performed in situ in the QCM cell by subsequently pumping the metal and linker solutions as well as pure ethanol through the QCM cell. For the first data point shown in Fig. 2 , the synthesis of the HKUST-1 SURMOF was interrupted after 30 cycles. The mass density of the synthesized SURMOF was determined to be 7.9 μg cm −2 , yielding a SURMOF thickness of 52 nm for a mass density of the ethanol-soaked HKUST-1 of 1.53 g cm −3 . Note that the density of the activated framework amounts to 0.98 g cm −3 (ref. 27 ), which has to be augmented by the density of ethanol contained in the pores. This value amounts to 0.56 g per 1 g HKUST-1 MOF [38] . After activating the sample at 65 °C in a flow of pure argon (with a flow rate is 100 ml min −1 ) overnight, the uptake of the guest molecules was studied again with the QCM. The initially pure argon was switched to an argon flow passing through liquid cyclohexane at room temperature (298 K), resulting in argon flow with a cyclohexane partial pressure of 130 mbar. The cyclohexane uptake by the 52-nm-thick HKUST-1 SURMOF is shown in Supplementary Fig. 3a . After the cyclohexane uptake experiments using the 52-nm-thick SURMOF film were performed, the SURMOF synthesis was continued in situ for additional 40 cycles. The sample thickness was recorded by QCM, resulting to an overall sample thickness of 110 nm (see Fig. 2 ). After activating the sample, the uptake of cyclohexane was studied (see Supplementary Fig. 3b ). Subsequently, the SURMOF synthesis was continued and the cyclohexane uptake was again investigated. In this way, the cyclohexane uptake by the HKUST-1 SURMOF was investigated for seven different thicknesses, that is, for film thicknesses of 52, 110, 190, 260, 340, 490 and 690 nm, see Supplementary Fig. 3 . The syntheses as well as the uptake experiments were performed at a temperature of 303 K. All uptake experiments were repeated at least twice for calculating the average value and the s.d. After all uptake experiments were completed, the sample quality was checked by out-of-plane XRD and scanning electron microscopy (SEM), see Supplementary Fig. 2 . The SEM images show a smooth and homogenous film without visible defects. It has to be stated that, at the experimental set-up, the volume in the QCM cell is 40 μl and the argon flow rate is 100 ml min −1 . It takes therefore ~0.024 s until the cyclohexane partial pressure in the QCM cell is established when switching from pure argon to cyclohexane-enriched argon. Hence, the time constants (see Fig. 3c ) are corrected by this value. How to cite this article: Heinke, L. et al. The surface barrier phenomenon at the loading of metal-organic frameworks. Nat. Commun. 5:4462 doi: 10.1038/ncomms5562 (2014).